On-chip steering of entangled photons in nonlinear photonic crystals One promising technique for working toward practical photonic quantum technologies is to implement multiple operations on a monolithic chip, thereby improving stability, scalability and miniaturization. The on-chip spatial control of entangled photons will certainly benefit numerous applications, including quantum imaging, quantum lithography, quantum metrology and quantum computation. However, external optical elements are usually required to spatially control the entangled photons. Here we present the first experimental demonstration of on-chip spatial control of entangled photons, based on a domain-engineered nonlinear photonic crystal. We manipulate the entangled photons using the inherent properties of the crystal during the parametric downconversion, demonstrating two-photon focusing and beam-splitting from a periodically poled lithium tantalate crystal with a parabolic phase profile. These experimental results indicate that versatile and precise spatial control of entangled photons is achievable. Because they may be operated independent of any bulk optical elements, domain-engineered nonlinear photonic crystals may prove to be a valuable ingredient in on-chip integrated quantum optics. During parametric downconversion, two lower-frequency photons (usually called the signal and idler) are generated from a pump photon via a nonlinear crystal. Due to the conservation of energy and momentum of the original pump photon, the frequency and momentum of the signal and idler are strongly correlated. In particular, the spatial entanglement of the photon pair has led to interesting research in many fields, including quantum imaging [1] , [2] , [3] , [4] , [5] , [6] , quantum lithography [7] , [8] , [9] , quantum metrology [10] , [11] , [12] , [13] and quantum computation [14] . To prepare specific two-photon states for various applications, the spatial entanglement of the signal and idler is tailored by manipulating the wavefront of the pump beam [15] , [16] or modifying the entangled photons after their generation [17] , [18] , [19] , using various optical elements, such as lenses, multi-slits or spatial light modulators. These bulk optical elements inevitably hinder the performance of the photonic quantum circuits during practical applications, which require more stability, scalability and miniaturization [20] , [21] , [22] , [23] , [24] . The aforementioned difficulty can be overcome with a different strategy that applies domain engineering in quadratic nonlinear photonic crystals, which is widely used in quasi-phase-matching (QPM) nonlinear optics [25] , [26] , [27] , [28] , [29] . Although the spatial control of entangled photons via domain engineering has been already theoretically proposed [30] , few related experiments, other than a recent experiment showing that the amplitude of the entangled photons can be modulated by a multi-stripe nonlinear photonic crystal [31] , have been attempted. Comprehensive control of spatial entanglement (particularly the phase of entangled photons) has still not been experimentally demonstrated. In this work, we experimentally demonstrate the steering of entangled photons (that is, the wavefront shaping of the entangled photons) via domain engineering in nonlinear photonic crystals. By introducing a transverse inhomogeneity into the crystal, the wavefront of the entangled photons can be shaped at will, and the propagation of the entangled photons can be steered. We investigate a periodically poled lithium tantalate (PPLT) crystal with a transverse parabolic phase profile and find that the generated entangled photons are focused at a fixed distance from the crystal. In this case, our engineered crystal is equivalent to a homogeneous nonlinear crystal and a focusing lens ( Fig. 1a ). Additionally, by translating the crystal, we realize a dual-focusing condition in which the two-photon is focused onto either of two symmetric directions. Under this condition, our engineered crystal serves as the entangled photon source, lens and beam splitter ( Fig. 1b ). 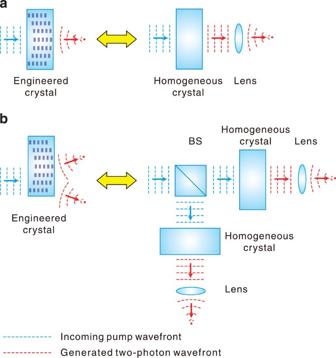Figure 1: The multifunction nonlinear photonic crystals. (a) In the single-focusing experiment, the engineered nonlinear photonic crystal serves as the entangled photon source and lens. (b) In the dual-focusing experiment, the engineered nonlinear photonic crystal serves as the entangled photon source, lens and beam splitter (BS). Figure 1: The multifunction nonlinear photonic crystals. ( a ) In the single-focusing experiment, the engineered nonlinear photonic crystal serves as the entangled photon source and lens. ( b ) In the dual-focusing experiment, the engineered nonlinear photonic crystal serves as the entangled photon source, lens and beam splitter (BS). Full size image Sample structure The quadratic nonlinear coefficient of our crystal is expressed as where d eff is the effective quadratic susceptibility, G m =2 m π/Λ is the m th-order reciprocal vector for the longitudinal modulation with period Λ in the beam's propagation direction z , F ( G m ) represents the corresponding Fourier coefficient and φ ( x ) and U ( x ) describe the nonuniform transverse phase and amplitude distributions, respectively. Because φ ( x )= ω p x 2 /(2 cfG 3 ) is parabolic, a two-photon carrying the phase front ω p x 2 /(2 cf ) is focused at a distance f from the crystal, where ω p is the angular pump frequency, c is the speed of light, G 3 is the third-order reciprocal vector that compensates for the longitudinal phase mismatching in the QPM and f represents the equivalent focal length of the crystal for the pump wavelength. The focusing behaviour can be described by the Huygens-Fresnel principle: each point on the primary wavefront acts as a source of secondary wavelets of the pump, as well as a source of the entangled photon pair. Therefore, such an engineered nonlinear photonic crystal is termed a QPM two-photon lens. By following the Huygens–Fresnel principle, we may engineer this crystal for any arbitrary spatial manipulation of entangled photons, such as focusing, beam-splitting or even multifunction integration. 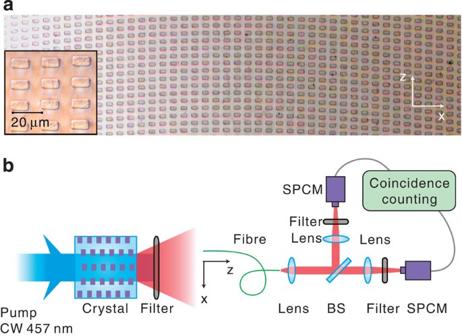Figure 2: Steering of the entangled photons by domain engineering. (a) Microscope photograph of the etched quadratic nonlinear crystal. The sample was fabricated from a congruent lithium tantalate crystal at room temperature by electric field poling technique. The periodicity in the longitudinal direction is Λ=13.917 μm, which ensures efficient entangled photon generation with the third-order reciprocal vectorG3=3×2π/Λ. The stripe interval is Λtr=20 μm, the stripe width isb=10 μm and the stripe length isL=6 mm. (b) Experimental setup. The crystal was pumped with a CW single longitudinal 457 nm laser. Degenerate photon pairs of 914 nm were generated at 180.1 °C with the polarization configuration ofe→e+e. After separation from the pump beam, the entangled photon pairs were directed into an optical fibre. Finally a 50/50 beam splitter (BS) was used, and photons on each path were collected by a lens and detected by a single-photon counting module (SPCM-AQR-14, PerkinElmer). A 10 nm bandwidth interference filter was placed before each detector to further suppress the pump photons. Figure 2a is a micrograph of our etched crystal. The transverse direction has a multi-stripe pattern that means that the amplitude modulation U ( x ) in equation (1) takes the form of a grating with a stripe width of 10 μm and a stripe interval Λ tr =20 μm. The initial position of each stripe follows the function ω p x 2 /(2 cfG 3 ), and the equivalent focal length of the crystal at the pump wavelength is designed to be f =33.3 mm. Figure 2: Steering of the entangled photons by domain engineering. ( a ) Microscope photograph of the etched quadratic nonlinear crystal. The sample was fabricated from a congruent lithium tantalate crystal at room temperature by electric field poling technique. The periodicity in the longitudinal direction is Λ=13.917 μm, which ensures efficient entangled photon generation with the third-order reciprocal vector G 3 =3×2π/Λ. The stripe interval is Λ tr =20 μm, the stripe width is b =10 μm and the stripe length is L =6 mm. ( b ) Experimental setup. The crystal was pumped with a CW single longitudinal 457 nm laser. Degenerate photon pairs of 914 nm were generated at 180.1 °C with the polarization configuration of e → e + e . After separation from the pump beam, the entangled photon pairs were directed into an optical fibre. Finally a 50/50 beam splitter (BS) was used, and photons on each path were collected by a lens and detected by a single-photon counting module (SPCM-AQR-14, PerkinElmer). A 10 nm bandwidth interference filter was placed before each detector to further suppress the pump photons. Full size image Single-focusing experiments The layout of our experiment is shown in Figure 2b . With the input tip of the fibre scanning in the transverse ( x ) and longitudinal ( z ) direction, we obtain the spatial correlation of entangled photon pairs by performing coincidence counting using the two detectors. The pump coincides with the centre of the parabolic PPLT sample. 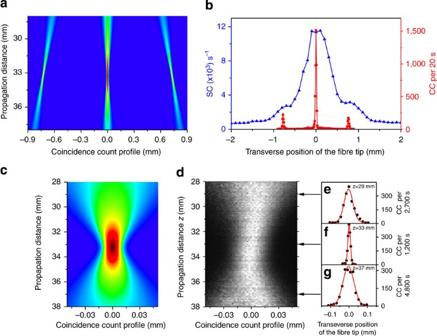Figure 3: The focused two-photon. (a) Simulation of the coincidence count profile as a function of the propagation distance. (b) Measured single (blue triangles) and coincidence (red dots) counts versus the transverse position of the fibre tip in the focal plane. (c) Simulation of the coincidence count profile around the focusing spot as a function of the propagation distance. (d) Measured coincidence count profile around the focusing spot as a function of the propagation distancez. Coincidence counts at each distance have been normalized respectively. (e–g) Measured transverse correlation at distances of 29, 33 and 37 mm, respectively. The solid red curves ine–gare Gaussian fittings. Figure 3a shows a simulation of the two-photon propagation dynamics based on the Huygens–Fresnel principle. Experimentally we obtained the minimum two-photon spatial correlation at a distance of z =33 mm, as can be seen in Figure 3b . The full width of the correlation peak, at which the intensity drops to 1/e 2 of its maximum value, was 28 μm. In contrast, we theoretically expected a 24-μm focusing spot with a full pump width of 0.82 mm in the experiment. The experimental value was slightly larger than the theoretical calculation primarily because the pump has a greater divergence angle than the TEM 00 mode. In addition to the primary focusing spot along the pump beam direction, which is located at x =0 mm, two other focusing spots were distributed symmetrically at x =+0.78 mm and −0.76 mm. The minor focusing spots resulted from multi-stripe interference. The theoretical separation between the two adjacent focusing spots was 2π cf /( ω p Λ tr )=0.76 mm, which is consistent with the experimental value. Figure 3: The focused two-photon. ( a ) Simulation of the coincidence count profile as a function of the propagation distance. ( b ) Measured single (blue triangles) and coincidence (red dots) counts versus the transverse position of the fibre tip in the focal plane. ( c ) Simulation of the coincidence count profile around the focusing spot as a function of the propagation distance. ( d ) Measured coincidence count profile around the focusing spot as a function of the propagation distance z . Coincidence counts at each distance have been normalized respectively. ( e – g ) Measured transverse correlation at distances of 29, 33 and 37 mm, respectively. The solid red curves in e – g are Gaussian fittings. Full size image Figure 3c shows an enlarged view of the simulated two-photon propagation dynamics around the focusing spot. Figure 3d shows the corresponding measured results. Whenever the fibre tip deviates from the focal plane, the measured two-photon spatial correlation widens. For example, at distances of z =29 mm and z =37 mm, the spatial correlation peak widths are 92 and 120 μm, respectively. The Rayleigh range is measured to be 0.9 mm. We used a TEM 00 Gaussian beam to fit the focusing behaviour and found that the two-photon behaves similar to a Gaussian beam with the pump wavelength (rather than the signal or idler wavelength). Dual-focusing experiments It is worth emphasizing that we engineered the parabolic PPLT with a transverse multi-stripe structure rather than a continuous structure. This introduces periodicity into the transverse direction of the crystal. For the structure that we fabricated, in any two stripes separated by a distance of 2π cf /( ω p Λ tr )=0.76 mm, the added phases of the entangled photon pairs are approximately equivalent. 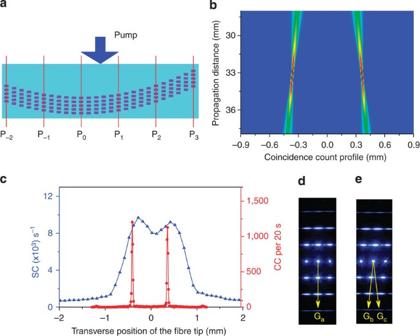Figure 4: The dual-focused two-photon. (a) The incident pump lies halfway between the two principal axes.Pj(j=0, ±1, ±2,...) are equivalent principal axes of the QPM two-photon lens. (b) Simulation of the coincidence count profile as a function of the propagation distance for the dual-focusing case. (c) Measured single (blue triangles) and coincidence (red dots) counts versus the transverse position of the fibre tip in the focal plane for the dual-focusing case. (d,e) Measured Fourier spectra of the multi-stripe parabolic PPLT for the single-focusing and dual-focusing case, respectively. The third-order reciprocal vectors used in the QPM are marked. Thus, the stripes at the 2 j π cf /( ω p Λ tr ) positions, where j is an integer, are all equivalent principal axes of the QPM two-photon lens, which are denoted by P j in Figure 4a . In our experiment, we find that when the crystal is translated in the x direction by multiples of 0.76 mm, the spatial distributions of the single counts and the two-photon coincidence counts remain identical. Figure 4: The dual-focused two-photon. ( a ) The incident pump lies halfway between the two principal axes. P j ( j =0, ±1, ±2,...) are equivalent principal axes of the QPM two-photon lens. ( b ) Simulation of the coincidence count profile as a function of the propagation distance for the dual-focusing case. ( c ) Measured single (blue triangles) and coincidence (red dots) counts versus the transverse position of the fibre tip in the focal plane for the dual-focusing case. ( d , e ) Measured Fourier spectra of the multi-stripe parabolic PPLT for the single-focusing and dual-focusing case, respectively. The third-order reciprocal vectors used in the QPM are marked. Full size image A new type of spatially entangled state is generated when the incident pump lies halfway between the two principal axes: this situation is illustrated in Figure 4a . The two-photon is deflected and focused onto either of the two symmetric directions around the pump beam. Figure 4b shows the simulated propagation dynamics of the dual-focused two-photon. Figure 4c shows the measured two-photon spatial correlation and single counts in the focal plane. There are two narrow correlation peaks with equivalent intensities, whereas the single counts follow a relatively smooth distribution. The measured peak interval of 0.77 mm agrees well with the theoretical prediction of 2π cf /( ω p Λ tr )=0.76 mm. The phase-matching of the dual focusing is actually achieved using two tilted reciprocal vectors as shown in Figure 4e . For such concurrent spontaneous parametric downconversion processes, it has been experimentally verified that their contributions to the two-photon state have a fixed phase relation [32] . Therefore, if we collect the photons in the two foci described here, we obtain a NOON state with N =2. As we change the incident position of the pump between the two principal axes, the proportions of the photon pairs focused onto the two directions can be dynamically tuned. In this case, the crystal serves as both the beam splitter (with a tunable splitting ratio) in the pump, and the lens. Phase matching analysis To obtain a better understanding of the working principle of the engineered crystal, we analysed the Fourier spectra of the multi-stripe parabolic PPLT, which are the measured far-field diffraction patterns of the crystal illuminated by the pump laser beam. Figure 4d corresponds to the single-focusing case, in which the pump coincides with the principal axis, whereas Figure 4e corresponds to the dual-focusing case, in which the pump beam lies halfway between the two principal axes. The third-order reciprocal vectors, which are used in the QPM, are marked by G a in Figure 4d and by G b and G c in Figure 4e . In the single-focusing case, G a ensures an efficient collinear downconversion and the two-photon is focused along the pump direction. In the dual focusing case, as G b and G c are not along the pump direction, the downconversion occurs using a non-collinear geometry. Hence, the two-photon is focused onto either of two possible directions, as shown in Figure 4c . We experimentally realized the on-chip steering of entangled photons, based on a domain-engineered nonlinear photonic crystal. Using a transversely parabolic PPLT, we demonstrated two-photon focusing and beam-splitting. Our measured results agree well with the designed parameters of the domain structure, which shows that accurate spatial control of entangled photons can be achieved via domain engineering. Because this approach enables the control of the amplitude and phase of the two-photon up to lithographic precision, unique optical elements, such as lenses with extremely small focal lengths and high numerical apertures, can be engineered. In our experiment, the crystal served as an entangled photon source, lens and beam splitter, as illustrated in Figure 1 . This multi-functionality shows the potential of integrating multiple optical transformations, such as a battery of lenses, into a single crystal. This multifunctional integration, which is inherent to the crystal, is free from any bulk optical elements and, therefore, may be exploited for on-chip integrated quantum optics. However, for a fully integrated device, other necessary functions (such as spectral filtering) should also be realized on the chip. This requires further consideration. The flexible, state-of-the-art crystal poling technique enabled the fabrication of a wide variety of domain structures, such that we could spatially control the entangled photons at will. Combined with the temporal control of the entangled photons using longitudinal domain engineering [33] , [34] , [35] , [36] , [37] , [38] , more interesting two-photon states may be prepared from nonlinear photonic crystals. This may attract interest in both fundamental physics and practical quantum technologies. Our technique might also find applications in research fields, such as quantum walk and continuous-variable encoding. Calculation of the two-photon correlation Assuming a monochromatic plane pump wave, the generated entangled two-photon state is where Ψ 0 is a normalization constant, Φ(Δ k z L )=sin(Δ k z L /2)/(Δ k z L /2) is the longitudinal detuning function (in which Δ k z = k p − k sz − k iz − G 3 and L is the stripe length), H tr is the transverse mode function (which is the Fourier transform of the transverse inhomogeneity, including the pump profile and the transverse domain structure), and are the transverse wave vectors of the signal and idler photons, respectively. For a transversely infinite and homogeneous crystal, the momentum correlation H tr is . However, in our experiment, a parabolic phase profile has been introduced, and therefore the momentum correlation of the photon pair is modified. According to Glauber's theory, the spatial correlation as a function of x and z can be derived to be where E 1 and E 2 are the electric fields evaluated at the two detectors and E p is the pump field. Equation (3) shows that the two-photon exhibits its minimum spatial correlation at a distance of z = f ; therefore the corresponding plane is termed the two-photon focal plane. For a transversely infinite and homogeneous crystal (that is, U ( x ′)=const.) in the focal plane, the two-photon spatial correlation is expressed as For a plane pump wave with an infinite beam width, the two-photon is focused onto an infinitesimal point. For a Gaussian pump beam, the two-photon is focused onto a spot, the size of which is determined by the pump beam size w 0 and the pump wavelength (rather than the signal or idler wavelength). How to cite this article: Leng, H. Y. et al . On-chip steering of entangled photons in nonlinear photonic crystals. Nat. Commun. 2:429 doi: 10.1038/ncomms1439 (2011).